Direct synthesis of single-walled aminoaluminosilicate nanotubes with enhanced molecular adsorption selectivity Internal functionalization of single-walled nanotubes is an attractive, yet difficult challenge in nanotube materials chemistry. Here we report single-walled metal oxide nanotubes with covalently bonded primary amine moieties on their inner wall, synthesized through a one-step approach. Conclusive molecular-level structural information on the amine-functionalized nanotubes is obtained through multiple solid-state techniques. The amine-functionalized nanotubes maintain a high carbon dioxide adsorption capacity while significantly suppressing the adsorption of methane and nitrogen, thereby leading to a large enhancement in adsorption selectivity over unfunctionalized nanotubes (up to four-fold for carbon dioxide/methane and ten-fold for carbon dioxide/nitrogen). The successful synthesis of single-walled nanotubes with functional, covalently-bound organic moieties may open up possibilities for new nanotube-based applications that are currently inaccessible to carbon nanotubes and other related materials. Single-walled nanotubes (‘SWNTs’) are important ‘building block’ materials for nanoscale science and technology, and have created great interest over the last two decades. Their one-dimensional geometry confers the potential for unique properties relevant to many applications [1] , [2] , [3] , [4] , [5] , [6] , [7] , [8] . Synthetic single-walled carbon nanotubes (CNTs), first prepared in 1991, are the most well-known SWNTs [1] . One of the main unsolved problems in CNT science is the covalent immobilization of functional moieties on their inner surfaces, which would allow a number of new ways to control the CNT properties and enable their use in ‘molecular recognition’ applications that exploit their 1-dimensional porosity (for example, catalysis, adsorption, membranes, sensors). The formation of covalent bonds at the CNT surface requires a transformation of carbon hybridization from sp 2 to sp 3 . This can be accomplished on the outer surface by several methods, albeit with rather harsh reaction conditions [2] , [3] , [4] . However, the concave interior surface of CNTs leads to an extremely high thermodynamic barrier for this transformation, due to which the interior surfaces of CNTs have been considered to be essentially unreactive [2] , [5] , [6] . Although several examples of infiltration of the CNT channel with various types of atomic, molecular or nanoparticle species have been reported [6] , [7] , [8] , as well as the modification of CNT tips with organic functional groups [2] , [9] , to date there is no demonstration of the interior functionalization of CNTs via the formation of covalent bonds. Recent work has indicated that the interior surface of CNTs may become reactive under certain extreme conditions, further corroborating the practically unreactive nature of CNT inner walls [10] , [11] . Synthetic metal oxide nanotubes could potentially overcome the above limitation of CNTs. More specifically, synthetic aluminosilicate and aluminogermanate SWNTs [12] , [13] , [14] , [15] , [16] have attracted substantial interest in recent years. This type of nanotube consists of an octahedral aluminium(III) hydroxide outer wall and a tetrahedral silanol inner wall, with doubly-coordinated hydroxyl groups on the outer wall and pendant hydroxyls on the inner wall ( Fig. 1a ). The chemistry of such nanotube materials, which is based upon aqueous-phase synthesis under mild (<100 °C) conditions, has advanced considerably over the last decade. Single-walled and double-walled aluminogermanate analogues of the aluminosilicate SWNTs have been synthesized [17] , [18] , [19] . Detailed molecular-level insights on the mechanism of formation of these nanoscopic objects have been obtained [18] , [20] , as well as the capability to engineer their shape and size with Ångstrom-level precision [21] . The first applications of these materials, for example, in the formation of high-quality polymer/nanotube membranes [22] and natural gas storage materials [23] have emerged recently. 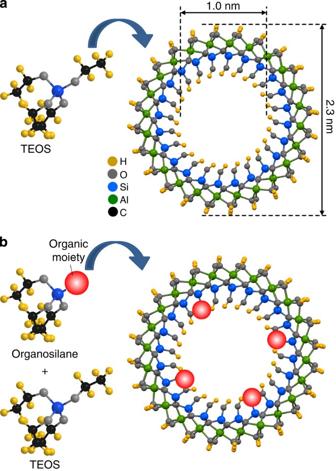Figure 1: Synthesis of aluminosilicate nanotubes. (a) Synthesizing bare aluminosilicate nanotubes using TEOS as the silicon source. (b) Forming nanotubes with organic moieties incorporated in their inner surfaces using a mixture of TEOS and a designed organosilane. Figure 1: Synthesis of aluminosilicate nanotubes. ( a ) Synthesizing bare aluminosilicate nanotubes using TEOS as the silicon source. ( b ) Forming nanotubes with organic moieties incorporated in their inner surfaces using a mixture of TEOS and a designed organosilane. Full size image The outer surfaces of the aluminosilicate SWNTs have been modified to a low degree via post-synthesis grafting with organosilane coupling agents [24] . However, this is a multi-step technique, which requires conversion of the aqueous SWNT gel into an anhydrous powder, and does not allow uniform distribution of the functionalizing agent along the length of the nanotube due to diffusion limitations induced by initial functionalization at the nanotube ends. These issues motivate the pursuit of a direct synthesis route for aluminosilicate SWNTs with organic functional groups immobilized at their interior surface. The key idea, as illustrated in Fig. 1b , is to (partially or completely) replace the siloxane reagent (Si-[O-R] 4 , usually tetraethyl orthosilicate (TEOS)) in the bare aluminosilicate SWNTs with an organosiloxane reagent (R'-Si-[O-R] 3 ). This ‘co-condensation’ approach has been successful in the preparation of organic-functionalized microporous [24] , [25] , [26] , [27] and mesoporous [28] , [29] silicate materials. However, its application to nanotubes has been much more difficult, likely owing to the unique mechanisms operating in the synthesis of these materials [20] , [21] . The first successful example of direct synthesis of organic-substituted aluminosilicate SWNTs involved the use of methyltriethoxysilane for producing methyl-functionalized aluminosilicate nanotubes [23] . However, the methyl group confers no additional functionality beyond increased hydrophobicity. Similar efforts using commercially available organosiloxane precursors with other functional groups (for example, aminopropyltriethoxysilane) have been unsuccessful. Here we describe a direct, template-free, synthesis route for preparing functional single-walled amine-functionalized aluminosilicate nanotubes (‘ANTs’) with up to 15% of the interior ≡Si-OH groups substituted by ≡Si-CH 2 NH 2 groups, via the use of a specifically synthesized precursor, aminomethyltriethoxysilane (AMTES). We hypothesize that the selection of the appropriate functional organosiloxane precursor is critical for the success of such an approach. Due to the small range of obtainable pore sizes (0.8–1 nm) of the SWNT and the confinement of the silanol groups in an ordered hydrogen-bonded network lining the pore [21] , we hypothesize that avoiding steric effects is important. For example, the smallest commercially available aminosiloxane precursor, aminopropyltriethoxysilane, is too bulky and hydrophobic, and therefore is found to not incorporate successfully into the nanotube structure. We design and synthesize a novel functional precursor (AMTES) which satisfies the required criteria and leads to successful incorporation into the nanotube wall to yield the ANT material. The structure, morphology and surface chemistry of ANTs are investigated by a range of solid-state characterization techniques, including conventional and cryogenic transmission electron microscopy (TEM/cryo-TEM), X-ray diffraction (XRD), nitrogen physisorption, elemental analysis, vibrational spectroscopy and solid-state NMR. The functionality of the primary amine groups in the interior of the SWNTs is assessed by CO 2 , CH 4 and N 2 adsorption. The amine-functionalized nanotubes show a dramatic improvement in CO 2 /CH 4 and CO 2 /N 2 adsorptive selectivity over the bare nanotubes (‘NTs’). The synthesis of amine-functionalized metal oxide SWNTs may facilitate a new class of functional SWNT materials obtainable by further chemical modifications of the amine groups. Morphology of amine-functionalized NTs The morphology of the ANTs is evaluated by conventional and cryogenic TEM ( Fig. 2 ). Low-resolution TEM images of both NTs and ANTs are shown in Fig. 2a . The ANTs show a smaller average length than the NTs (the average length of NT is 160 nm and of ANT 50 nm). The higher-resolution cryo-TEM images of NTs and ANTs ( Fig. 2b ) confirm the nanotubular structure of both materials. Electron diffraction (ED) was employed to investigate the crystallinity along the axis of NTs and ANTs ( Fig. 2c ). The ED patterns from both ANT and NT samples show an ordered nanotube wall structure. However, the NT reflections (006), (071) and (002) become less sharp, and reflections (004) and (063) are very weak or absent in the ED pattern of ANTs. The ED pattern from the post-synthesis functionalized nanotubes ( Supplementary Fig. 1 ) [30] , in which the organic moieties are likely immobilized at the pore mouth, is nearly identical to the pattern from the bare NT. These observations indicate successful random substitution of AMTES in the nanotube inner wall. 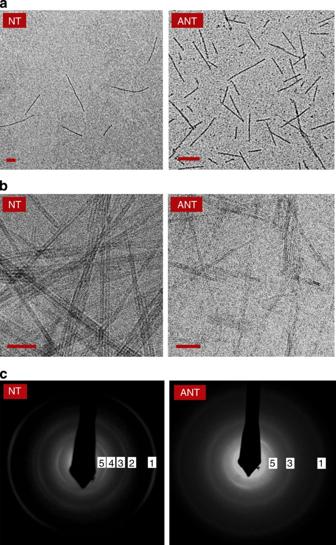Figure 2: Characterization of NTs and ANTs by TEM and ED. (a) Conventional and (b) cryo-TEM images. (c) ED patterns of NTs and ANTs. The scale bar for the conventional TEM images represents 20 nm, and for cryo-TEM images 10 nm. The reflections numbered 1–5 in the ED patterns are assigned to (006), (004), (063), (071) and (002).14 Figure 2: Characterization of NTs and ANTs by TEM and ED. ( a ) Conventional and ( b ) cryo-TEM images. ( c ) ED patterns of NTs and ANTs. The scale bar for the conventional TEM images represents 20 nm, and for cryo-TEM images 10 nm. The reflections numbered 1–5 in the ED patterns are assigned to (006), (004), (063), (071) and (002). [14] Full size image Interior surface properties The interior surface properties of the ANTs are comprehensively evaluated by a combination of N 2 physisorption, 13 C solid-state NMR, Fourier transform (FT)-Raman spectroscopy and elemental analysis. N 2 physisorption is an excellent tool to estimate the expected pore volume reduction due to the AMTES substitution for the ANT synthesis. The raw physisorption isotherms and the deduced pore size distributions and micropore surface areas are presented in Fig. 3 . The lower pore volume of ANTs and the occurrence of the maximum in the pore size distribution at a smaller pore size (8.7 Å for ANTs versus 9.5 Å for NTs), are both due to the larger size of the immobilized ≡Si-CH 2 NH 2 group in comparison with the ≡Si-OH group in the NTs. Given the volumes of the hydroxyl and the aminomethyl groups (16.9 and 38.1 Å 3 , as estimated from the atomic van der Waals radii), the fractional organic substitution ratio in the ANTs can be calculated by comparing the micropore volumes of the NTs and ANTs. The derived fractional organic substitution is 0.16, which is close to the AMTES:TEOS ratio (0.2) used in the ANT synthesis. The atomic compositions derived from elemental analysis are summarized in Supplementary Table 1 , and the raw elemental analysis data are presented in Supplementary Table 2 . First, the identical Si:Al ratio (0.5) in both the ANTs and NTs rules out the presence of impurities caused by possible self-polymerization of AMTES and TEOS during the synthesis. Second, the nitrogen and carbon signals are only observed in ANTs, thereby showing the presence of the organic moieties in the sample. The fractional organic substitution estimated from the carbon signal is 0.16, and from the nitrogen signal is 0.11, broadly consistent with the quantification from N 2 physisorption (0.16). 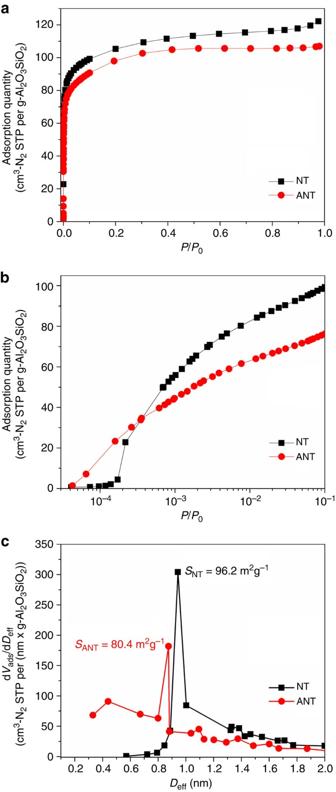Figure 3: Porosity characterization of NTs and ANTs using N2physisorption. (a) Full isotherms on a linear scale. (b) Isotherms on semilog scale to highlight the low-pressure region. (c) Pore size distributions andt-plot micropore surface areas derived from the physisorption isotherms. Figure 3: Porosity characterization of NTs and ANTs using N 2 physisorption. ( a ) Full isotherms on a linear scale. ( b ) Isotherms on semilog scale to highlight the low-pressure region. ( c ) Pore size distributions and t -plot micropore surface areas derived from the physisorption isotherms. Full size image Although N 2 physisorption and elemental analysis suggest the presence of immobilized organic moieties in the ANT, 13 C solid-state NMR and FT-Raman spectroscopy identify the organic species. The single peak at 27 p.p.m. in the 13 C NMR spectrum ( Fig. 4a ) of the ANT is assigned to the aminomethyl group. The absence of peaks from the ethoxy groups (57 p.p.m. for -OCH 2 - and 17 p.p.m. for -CH 3 ) [31] of the reagent AMTES provides clear support for the success of the ANT synthesis. When using TEOS for NT synthesis, the ethoxy groups are hydrolysed and a Q 3 (6Al) ≡Si-OH coordination environment is formed [15] , [20] , [30] . This coordination is exclusively found in the aluminosilicate NT material. An identical hydrolysis of ethoxy groups and formation of an equivalent T 3 (6Al) ≡Si-CH 2 NH 2 environment [15] , [30] is clear evidence of the formation of the aminomethylsilane-substituted single-walled aluminosilicate NTs (ANTs). The FT-Raman spectra for both NTs and ANTs are shown in Fig. 4b . The additional peaks (1,298, 1,450, 1,506 and 2,950 cm −1 ) seen in the ANT material, in comparison with the NT material, are assigned to C-N stretching, C-H deformation, C-N deformation and C-H stretching vibrations, respectively [32] . These vibrational modes further confirm the presence of the aminomethyl groups in the ANT material. 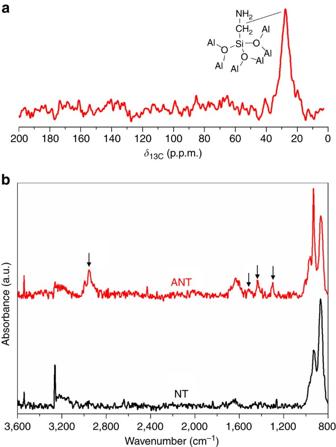Figure 4: Interior surface properties of NTs and ANTs. (a)13C solid-state NMR spectrum of ANT. (b) FT-Raman spectra of NT and ANT. The arrows identify peaks assigned to C-N and C-H vibrations in the ANT sample. Figure 4: Interior surface properties of NTs and ANTs. ( a ) 13 C solid-state NMR spectrum of ANT. ( b ) FT-Raman spectra of NT and ANT. The arrows identify peaks assigned to C-N and C-H vibrations in the ANT sample. Full size image Silicon coordination The Si coordination in the ANTs is rigorously assessed by 29 Si and 27 Al NMR. 29 Si direct polarization NMR spectra are shown in Fig. 5a . For both NTs and ANTs, the peak at −79 p.p.m. is known as the Q 3 (6Al) ≡Si-OH fingerprint [15] , [20] , [30] and originates from the use of TEOS as a Si source in both cases. The peak at −57 p.p.m., observed only in ANTs but not in NTs, occurs from the additional Si source (AMTES) used in ANT synthesis. According to the aforementioned discussion regarding the absence of the ethoxy groups, the peak at −57 p.p.m. could be assigned to either T 3 (3Si) or T 3 (6Al) Si, wherein T 3 (3Si) would be due to self-polymerization of AMTES and T 3 (6Al) would be the fingerprint of isolated aminomethlysilane groups in the ANTs. To differentiate between these two possibilities, a control experiment was performed by immobilization of AMTES on a mesoporous silica support (SBA-15), resulting in a combination of T 1 (1Si), T 2 (2Si), and T 3 (3Si) coordination (the raw 29 Si NMR spectrum is shown in Supplementary Fig. 2 ). The 29 Si chemical shift of the T 3 (3Si) silicon was found at −72 p.p.m., which is quite different from the −57 p.p.m. chemical shift seen in the ANTs. Hence, the peak at −57 p.p.m. is very likely due to the isolated ≡Si-CH 2 NH 2 aminomethylsilane groups in the ANTs. Another supporting evidence for the peak assignment is that when using methytriethoxysilane (MTES) as the reagent, there is only a 2 p.p.m. difference between the T 0 (neat reagent in solution state, −41 p.p.m.) and T 3 (6Al) ≡Si-CH 3 peak (isolated methylsilane groups in the NT, −43 p.p.m.) [23] . In our AMTES system ( Supplementary Table 3 ), a similar 2 p.p.m. difference is also observed for T 0 (−55 p.p.m., Supplementary Fig. 3 ) and T 3 (6Al) (−57 p.p.m.). Provided that the repetition delay is chosen to be long enough, the integrated areas under the −57 p.p.m. and −79 p.p.m. Si peaks in the direct polarization NMR spectrum can be used for quantifying the fractional substitution of ≡Si-CH 2 NH 2 for ≡Si-OH groups. For the ANT sample, this quantity is determined to be 0.18. The 27 Al spectra of NTs and ANTs are nearly identical ( Fig. 5b ). The peak at −4 p.p.m. is due to the octahedral Al coordination in both nanotubes. The quantification of the fractional substitution of T 3 (6Al) for Q 3 (6Al) by various techniques is shown in this work ( Supplementary Table 4 ). The average fractional substitution from all the analytical techniques is 0.15. The fractional substitution derived from the elemental analysis represents the organic moiety immobilized on both interior and external surface of ANTs whereas the values deduced from the 29 Si solid-state NMR and N 2 physisorption represent the amine moiety grafted only on the interior surface of ANTs. 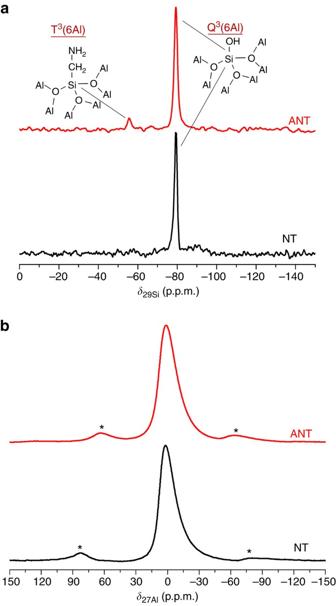Figure 5: Solid-state NMR spectra of NTs and ANTs. (a)29Si direct polarization and (a)27Al solid-state NMR spectra of NTs and ANTs. The asterisks denote the spinning side bands. Figure 5: Solid-state NMR spectra of NTs and ANTs. ( a ) 29 Si direct polarization and ( a ) 27 Al solid-state NMR spectra of NTs and ANTs. The asterisks denote the spinning side bands. Full size image To gain more insight into the connectivity between Si (from both TEOS and AMTES as Si sources) and Al atoms in the ANT wall, 29 Si/ 27 Al transfer of populations in double resonance (TRAPDOR) experiments were employed [33] . The TRAPDOR technique directly probes the dipolar coupling between a spin=1/2 nucleus ( 29 Si) and a spin>1/2 nucleus ( 27 Al), and thereby characterizes the proximity of these two nuclei [33] , [34] . Practically speaking, in the presence of a dephasing pulse from the 27 Al channel, the 29 Si peak intensity will be reduced if the Si atoms are within a few Angstroms of the Al atoms [33] , [34] . The TRAPDOR spectra for the ANT are shown in Fig. 6 . A clear intensity reduction is observed for both Q 3 (6Al) and T 3 (6Al) peaks in the presence of the 27 Al dephasing pulse, confirming the close proximity between Al and Si atoms and therefore our peak assignment. On the other hand, a control sample composed of a physical mixture of mesoporous silica (SBA-15) and α-alumina is also measured ( Supplementary Fig. 4 ). No intensity reduction of the Si signal is observed due to a lack of silicon-aluminium connectivity. 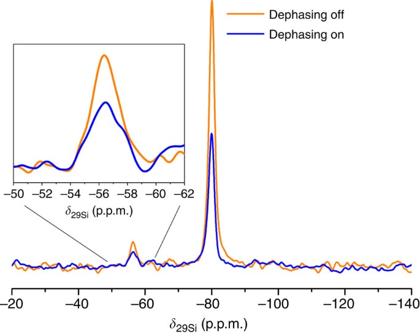Figure 6:29Si/27Al TRAPDOR NMR spectra of the ANT material. The two spectra obtained from the29Si/27Al TRAPDOR sequence in the presence (blue) and absence (orange) of the dephasing pulse. Figure 6: 29 Si/ 27 Al TRAPDOR NMR spectra of the ANT material. The two spectra obtained from the 29 Si/ 27 Al TRAPDOR sequence in the presence (blue) and absence (orange) of the dephasing pulse. Full size image Structural modelling On the basis of the interior surface chemistry and framework characterizations, a structural model of the ANT was constructed ( Fig. 7a ). Using the structural models of the NT and ANT materials, XRD simulations were then performed. The comparison of the simulated and experimental XRD patterns for NTs and ANTs is summarized in Fig. 7b . As discussed in our previous works [15] , [22] , the XRD patterns for NTs are not dominated by Bragg diffraction but by scattering from small bundles of NTs. In particular, both computational and experimental evidence shows that the NTs form small bundles of three or four individual nanotubes. The XRD pattern is fully explained by the scattering form factor of a bundle composed of three or four tubular objects [35] . The immobilization of the aminomethyl groups at the inner surface of the nanotubes causes a deviation in the form factor from the plain NTs, which describes an ideal core-shell cylindrical object with uniform scattering length density. This subtle difference between NTs and ANTs is successfully captured in both experimental and simulated XRD patterns, wherein the ANT shows less prominent features in the regions of 5–6°, 8–10° and 12–14° 2 θ . The excellent agreement between experimental and computational XRD patterns for ANT further demonstrates the successful synthesis of ANTs. Although nanotube synthesis with 20% AMTES substitution for TEOS successfully yielded ANTs with 15% T 3 (6Al) substitution for Q 3 (6Al) in the nanotube wall, we are so far unable to synthesize ANTs with 50 and 100% AMTES substitution ( Supplementary Figs 5–7 ). To further advance the synthesis of organic-functionalized single-walled metal oxide NTs, a better understanding of the molecular-level events occurring during the synthesis is necessary [20] , [21] . 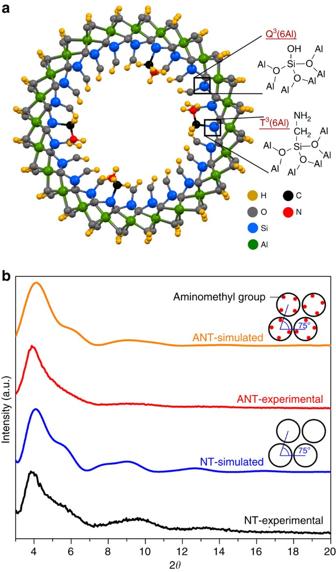Figure 7: Structural model and XRD simulations of NTs and ANTs. (a) Proposed structural model of ANT. (b) Measured and simulated XRD patterns of NTs and ANTs. Figure 7: Structural model and XRD simulations of NTs and ANTs. ( a ) Proposed structural model of ANT. ( b ) Measured and simulated XRD patterns of NTs and ANTs. Full size image Gas adsorption Single-component gas adsorption measurements via quartz crystal microbalance-based techniques [36] were performed to evaluate the functionality of the ANT material. The CO 2 /N 2 and CO 2 /CH 4 molecular pairs were chosen to assess the effect of the aminomethyl groups on adsorptive selectivity for CO 2 , which is relevant to carbon capture from flue gas and natural gas purification [37] , [38] . The full adsorption isotherms are shown in Fig. 8 , and the ideal adsorption selectivity of NTs and ANTs is summarized in Fig. 9 . In this work, the ideal adsorption selectivity is defined in the standard manner, as the ratio of the single-component adsorption uptakes of two different adsorbate molecules at the same partial pressure. As shown in Fig. 9 , ANTs with a 15% aminomethyl group substitution for hydroxyls exhibit a dramatic improvement in selectivity over the bare NTs for both CO 2 /CH 4 (up to four-fold increase) and CO 2 /N 2 (up to ten-fold increase). 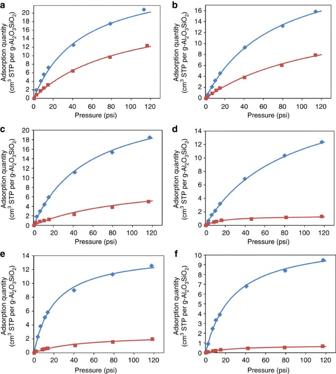Figure 8: CO2and CH4adsorption isotherms of NT and ANT materials. The adsorption isotherms of (a) CO2at 25 °C, (b) CO2at 67 °C, (c) CH4at 25 °C, (d) CH4at 67 °C, (e) N2at 25 °C and (f) N2at 67 °C for NT (blue diamonds) and ANT (red squares); and the fitted curves (solid lines) to the Langmuir model. Figure 8: CO 2 and CH 4 adsorption isotherms of NT and ANT materials. The adsorption isotherms of ( a ) CO 2 at 25 °C, ( b ) CO 2 at 67 °C, ( c ) CH 4 at 25 °C, ( d ) CH 4 at 67 °C, ( e ) N 2 at 25 °C and ( f ) N 2 at 67 °C for NT (blue diamonds) and ANT (red squares); and the fitted curves (solid lines) to the Langmuir model. 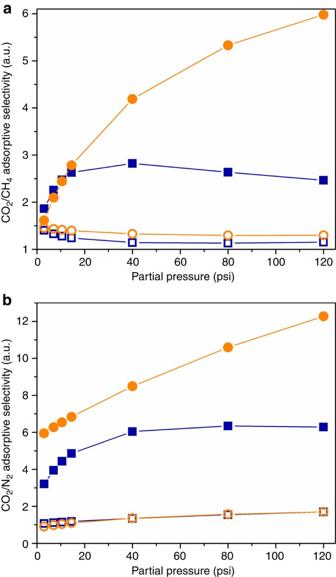Figure 9: Ideal CO2adsorption selectivity of NT and ANT materials. Ideal CO2adsorption selectivity of NTs (open symbols) and ANTs (closed symbols), for gas pairs of (a) CO2/CH4and (b) CO2/N2, at 25 °C (squares) and 67 °C (circles). Full size image Figure 9: Ideal CO 2 adsorption selectivity of NT and ANT materials. Ideal CO 2 adsorption selectivity of NTs (open symbols) and ANTs (closed symbols), for gas pairs of ( a ) CO 2 /CH 4 and ( b ) CO 2 /N 2 , at 25 °C (squares) and 67 °C (circles). Full size image To gain more insight into the observed selectivity enhancements and evaluate the affinity of the ANT and NT walls for the adsorbate molecules, the Henry’s constants for adsorption in each nanotube material were obtained from fits of the full isotherms to the Langmuir model ( Supplementary Note 1 ). The Henry’s constant ratios between ANTs and NTs ( K ANT /K NT ) are summarized in Supplementary Table 5 . The detailed Langmuir fitting parameters are presented in Supplementary Table 6 . In general, the Henry’s constants decrease for all the adsorbates when partially replacing surface hydroxyl groups with aminomethyl groups. As expected, the isolated aminomethyl (≡Si-CH 2 NH 2 ) groups in the ANTs possess overall weaker affinities for the adsorbates in comparison with the hydroxyl (≡Si-OH) groups. However, the aminomethyl groups greatly suppress the adsorption of CH 4 and N 2 in relation to CO 2 , thereby leading to a large enhancement in CO 2 /CH 4 and CO 2 /N 2 adsorption selectivity. Furthermore, the relative suppression in CH 4 and N 2 adsorption becomes more efficient when the temperature is increased from 25 °C to 67 °C, as well as by increasing the pressure, thereby leading to increased adsorption selectivity with both temperature and pressure. Previous computational and experimental works suggest that single-walled carbon nanotubes of comparable diameter (~1 nm) have a maximum CO 2 /CH 4 and CO 2 /N 2 adsorption selectivity of about 7 at 25 °C and a low pressure of 1 atm, with the selectivity declining as pressure increases, for example, to about 5.5 at 8 bar (~120 psi) [39] , [40] . More importantly, in the case of carbon nanotubes there is no available route for controlling these properties by functionalizing or modifying their interior surfaces. The smaller reduction of Henry’s constant for CO 2 is due to the mechanism of amine group binding to CO 2 molecules. It is well known that one equivalent of a free base moiety—typically water—is needed for a primary amine to adsorb one equivalent of CO 2 [41] , [42] . However, under anhydrous conditions such as in the present adsorption measurements, two adjacent primary amines are required to adsorb one equivalent of CO 2 . The primary amine groups are expected to be distributed in a random manner at the inner surface of the ANTs, and there is no evidence available for preferred clustering (or non-clustering) of the aminomethylsilane functional sites. At a 15% substitution of silanol groups by aminomethyl groups in the confined space of the inner nanotube wall, we expect the presence of isolated amine sites as well as amine groups in close proximity to each other. Given the adsorption mechanisms discussed above, amine groups in close proximity will provide a positive contribution to CO 2 adsorption, whereas an isolated amine would likely show lower CO 2 affinity than the surface hydroxyls. These two competing effects, present only for CO 2 adsorption but not for CH 4 and N 2 , are likely to be the key factor leading to a relatively small reduction of Henry’s constant for CO 2 and the high CO 2 /CH 4 and CO 2 /N 2 selectivity in ANTs. In conclusion, through a single-step approach, we have successfully synthesized single-walled aminoaluminosilicate nanotubes (ANTs) with a 15% aminomethyl group substitution for the hydroxyl groups on the interior nanotube wall. A combination of characterization techniques including TEM, cryo-TEM, 13 C, 29 Si and 27 Al solid-state NMR, FT-Raman spectroscopy, elemental analysis, nitrogen physisorption and XRD measurements and simulations, have yielded conclusive structural information on the ANTs at the molecular level. CO 2 , CH 4 and N 2 adsorption measurements on the bare NTs and amine-functionalized ANTs have demonstrated that the interior surface properties can be significantly tailored by the incorporation of the primary amines. The modified interior surface results in dramatically enhanced CO 2 /CH 4 and CO 2 /N 2 ideal adsorption selectivity. This work elucidates the fabrication of functionalized single-walled metal-oxide nanotube materials with altered interior surface properties. Such an approach to synthesize functional nanotube materials can enable a wider range of applications for nanotubes, which have so far been inaccessible to other nanotube systems such as carbon nanotubes. Synthesis of aminomethyltriethoxysilane AMTES was synthesized by treating the commercially available chloromethyltriethoxysilane with gaseous ammonia using a Parr reactor. The reaction was performed anhydrously at 900–1,000 psi and 100 °C for 5 h. The synthesis details were identical to that described in our previous work. [43] Nanotube synthesis TEOS and AMTES were mixed with aluminium-tri-sec-butoxide in a glove box filled with nitrogen. The mixture, with a TEOS:AMTES:Al:HClO 4 molar ratio of (1− x ): x :2:1, was added into a Teflon jar (1,000 ml capacity) containing 500 ml of 38 mM perchloric acid. Bare aluminosilicate nanotubes (‘NTs’) were obtained when x =0; whereas ANTs were synthesized when x =0.2. Synthesis products with x =0.5 and 1 are discussed in the Supplementary Figs 5–7 . The aqueous mixture was vigorously stirred at room temperature in ambient conditions for 24 h. The solution was then diluted with deionized water water by a factor of 3.8 with respect to volume, and then stirred at 95 °C for 96 h. Once the temperature was brought to 95 °C, the solution turned from cloudy to clear in about 1 h. After the solution was cooled to room temperature, a 30 wt% ammonia solution was added dropwise until gelation of the suspended nanotubes occurred. The gel was isolated by centrifugation at 7,000 r.p.m. for 10 min. The supernatant was discarded and a few drops of 10 N hydrochloric acid were added to the gel, thereby re-dispersing the nanotubes. The gel was dialyzed against 10 wt% ammonium hydroxide solution for 24 h and then against deionized water water for 3 days, using a dialysis membrane with a 15 kDa molecular weight cutoff. To obtain powder samples, the purified gel was dried at 60 °C and then ground lightly to disperse the agglomerated nanotubes. Approximately 1 g of powder sample is obtained from a 1 l synthesis batch volume. Transmission electron microscopy TEM images were collected using a JEOL JEM-2200FS 200 kV field emission transmission electron microscope with an in-column Omega energy filter (operated at 200 kV). Detailed sample preparation procedures are described in our previous work [21] . Cryo-TEM images were recorded at the Apkarian Integrated Electron Microscopy Core (Emory University) using a JEOL JEM-1210 microscope operated at 100 kV [15] . X-ray diffraction measurements and simulations XRD measurements in Bragg–Brentano geometry were performed on a PAnalytical X’pert Pro MPD diffractometer operating with a Cu Kα source. Diffraction data were collected with a collimator and proportional (Miniprop) He-filled detector, in the range of 3–30° 2 θ and a step size of 0.05° 2 θ . The Reflex module of the Materials Studio 3.2 package (Accelrys) was used for XRD pattern simulations, and the methodological details have been reported in our previous work [15] . Nitrogen physisorption Nitrogen physisorption measurements were carried out on a Micromeritics Tristar II at 77 K. The sample was placed in an analysis tube and degassed under 15 mTorr at 200 °C for 12 h before physisorption measurements. Solid-state NMR The 13 C, 27 Al and 29 Si MAS NMR measurements were carried out on a Bruker DSX 300 using a 7 mm rotor. For 13 C cross-polarization MAS NMR, the sample was spun at 5 kHz, and a single π /2 pulse with a duration of 5 μs and a repetition time of 4 s was used. The sample was spun at 5–6 kHz for 27 Al MAS NMR, for which a single pulse of π/6 (duration 0.6 μs) and a repetition time of 0.1 s was used. For 29 Si MAS NMR, direct polarization scans were performed with repetition times of 10 s at π /2 single pulse (duration 5 μs) and 5 kHz spinning rate. The chemical shifts of 13 C, 27 Al and 29 Si were referenced to adamantane ( 13 C chemical shift at 38.45 p.p.m. ), an aqueous solution of aluminium trichloride ( 27 Al chemical shift at 0 p.p.m. ), and solid 3-(trimethylsilyl)-1-propanesulphonic acid sodium salt ( 29 Si chemical shift at 0 p.p.m. ), respectively. The 29 Si/ 27 Al Transfer of Populations in Double Resonance (TRAPDOR) NMR experiments were carried out on a Bruker Avance III 400 using a triple resonance probe equipped for 3.2 mm MAS rotors. The pulse sequence followed the previous literature using decoupling of the 27 Al-nucleus during the evolution period [33] . The MAS spinning speed was set to 5 kHz. A dephasing time of 2 ms (10 rotor periods) was applied for the 27 Al decoupling with a frequency of ~100 kHz. Raman spectroscopy FT-Raman spectra were obtained on a Bruker Vertex 80v spectrometer with dual FTIR and FT-Raman benches and CaF 2 beamsplitter. Elemental analysis was performed by Columbia Analytical Services, Inc. Gas adsorption measurements Adsorption measurements were performed with a quartz crystal microbalance-based measurement apparatus developed in-house [36] . For the sample preparation, the as-synthesized NT or ANT gel was drop-coated by depositing a few drops on the quartz crystal microbalance substrate. The substrates were then pre-baked in an oven at 110 °C and atmospheric pressure for 30 min. The samples were then mounted in the measurement apparatus and degassed in situ at 180 °C and 4 mTorr for about 24 h before adsorption measurements. Single-component adsorption isotherms of CO 2, CH 4 and N 2 in the two types of NTs were then collected at 25 °C and 67 °C and pressures ranging from 0.3–120 psi (about 8 atm). Measurements were taken in pressure intervals of 2–3 psi (below 1 atm) and ~40 psi (above 1 atm). How to cite this article: Kang, D.-Y. et al. Direct synthesis of single-walled aminoaluminosilicate nanotubes with enhanced molecular adsorption selectivity. Nat. Commun. 5:3342 doi: 10.1038/ncomms4342 (2014).